Evolution of interlayer coupling in twisted molybdenum disulfide bilayers Van der Waals coupling is emerging as a powerful method to engineer physical properties of atomically thin two-dimensional materials. In coupled graphene–graphene and graphene–boron nitride layers, interesting physical phenomena ranging from Fermi velocity renormalization to Hofstadter’s butterfly pattern have been demonstrated. Atomically thin transition metal dichalcogenides, another family of two-dimensional-layered semiconductors, can show distinct coupling phenomena. Here we demonstrate the evolution of interlayer coupling with twist angles in as-grown molybdenum disulfide bilayers. We find that the indirect bandgap size varies appreciably with the stacking configuration: it shows the largest redshift for AA- and AB-stacked bilayers, and a significantly smaller but constant redshift for all other twist angles. Our observations, together with ab initio calculations, reveal that this evolution of interlayer coupling originates from the repulsive steric effects that leads to different interlayer separations between the two molybdenum disulfide layers in different stacking configurations. Vertically stacked two-dimensional (2D) atomic layers have attracted immense research interest recently. In graphene bilayers and graphene/boron nitride heterostructures, for example, the weak van der Waals (vdW) interaction leads to new physical phenomena ranging from new van Hove singularities [1] , [2] , [3] , [4] and Fermi velocity renormalization [5] , [6] to unconventional quantum Hall effects [7] and Hofstadter’s butterfly pattern [8] , [9] , [10] , [11] , [12] . In gapless graphene, the interlayer coupling depends sensitive on the interlayer twist angle, and the electronic properties around the K point is modified the most when the twist angle is small [5] , [6] . However, the evolution of interlayer coupling in gapped 2D materials, such as the 2D transition metal dichalcogenides [13] , [14] , can be very different. In this article, we use MoS 2 bilayers as a model system to investigate the evolution of interlayer coupling with the twist angle in 2D transition metal dichalcogenide semiconductors. Monolayer MoS 2 exhibits many intriguing physical properties, including a direct optical bandgap of ~1.8 eV in the visible range [15] , [16] , a strong exciton binding energy [17] and valley selective circular dichroism [18] , [19] , [20] that make it a promising material for next-generation nano-electronics [21] , photonics [22] , photovoltaics [23] and valleytronics [18] , [19] , [20] . Previous studies on naturally AB-stacked MoS 2 bilayers show that the weak interlayer couplings can significantly modify the physical properties [24] , [25] , but little is known on how they evolve with the twist angle in arbitrarily stacked MoS 2 bilayers. Here we present the first study on the interlayer coupling in as-grown MoS 2 bilayers with different stacking configurations and reveal an unexpected evolution of the vdW coupling with twist angles. We find that the indirect bandgap size and the out-of-plane phonon vibrational frequency of MoS 2 bilayers vary appreciably with the twist angle. Such variations are rooted in the repulsive steric effect, which in turn determines the interlayer distance between MoS 2 bilayers. Twisted MoS 2 bilayer sample In our experiment, we grow triangle-shaped MoS 2 monolayers and bilayers with different stacking orders by chemical vapour deposition (CVD). Our growth is based on the recent progress in MoS 2 monolayer synthesis [26] , [27] , [28] but with modified growth conditions (see Methods section). Our key control is to decrease the nucleation rate at the initial stage of growth to make the vertical layer-by-layer growth mode preferable. We can grow MoS 2 bilayers on various substrates, including mica, fused silica and SiO 2 /Si with yield as high as 30%. (The other 70% are mainly monolayers). 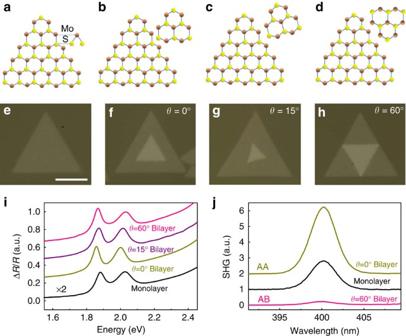Figure 1: Twisted MoS2bilayers. (a–d) Schematics of the atomic structure of a MoS2monolayer (a) and bilayers with twist angles ofθ=0° (b),θ=15° (c) andθ=60° (d). (e–h) Optical reflection images of a MoS2monolayer and twisted bilayers corresponding to (a–d). Scale bar, 10 μm. (i) Difference reflection spectra (ΔR/R) from the monolayer and bilayers corresponding toe–h. The two resonance peaks are characteristics of direct exciton transitions in MoS2. (j) Second-harmonic generation (SHG) signal from a MoS2monolayer, an AA-stacked bilayer (θ=0°) and an AB-stacked bilayer (θ=60°). The traces ini,jare shifted vertically for clarification. Figure 1e–h show, respectively, optical reflection images of a monolayer and bilayers with twist angles of θ =0°, 15° and 60° on fused silica substrates. In bilayer samples, the smaller top layer is above the larger bottom layer, leading to a doubled optical contrast. Reflection spectra ( Fig. 1i ) of the samples show prominent resonances at 1.85 and 2.05 eV, characteristic of the direct exciton transitions in MoS 2 layers. Figure 1: Twisted MoS 2 bilayers. ( a – d ) Schematics of the atomic structure of a MoS 2 monolayer ( a ) and bilayers with twist angles of θ =0° ( b ), θ =15° ( c ) and θ =60° ( d ). ( e – h ) Optical reflection images of a MoS 2 monolayer and twisted bilayers corresponding to ( a – d ). Scale bar, 10 μm. ( i ) Difference reflection spectra (Δ R / R ) from the monolayer and bilayers corresponding to e – h . The two resonance peaks are characteristics of direct exciton transitions in MoS 2 . ( j ) Second-harmonic generation (SHG) signal from a MoS 2 monolayer, an AA-stacked bilayer ( θ =0°) and an AB-stacked bilayer ( θ =60°). The traces in i , j are shifted vertically for clarification. Full size image The twist angle of MoS 2 bilayer can be readily determined through the relative orientation of the top and bottom triangle shapes. In MoS 2 , each Mo atom is covalently bonded to six S atoms in a trigonal prismatic arrangement ( Fig. 1a ), and the triangle-shaped layers have been shown to terminate with Mo at zigzag edges in scanning tunnelling microscopy [29] , transmission electron microscopy [28] and ab initio theoretical studies [30] . Therefore, the orientation of each triangle is directly correlated with the microscopic crystal orientation of the MoS 2 layer, and we can determine the twist angle of a MoS 2 bilayer from the relative rotation of the two vertically stacked triangles ( Fig. 1b–d ). We further confirmed the AA-stacking order in θ =0° bilayers and the AB-stacking order in θ =60° bilayers using second-harmonic generation (SHG) measurements ( Fig. 1j ), where SHG signal is strongly suppressed for AB-stacked bilayer owing to its overall inversion symmetry [31] ( Supplementary Note 1 ). Interlayer electronic coupling evolution in MoS 2 bilayers The interlayer interaction can significantly modify both the electronic band structure and phonon vibrations in MoS 2 bilayers. We first investigate the evolution of the electronic coupling in different twisted MoS 2 bilayers using photoluminescence (PL) spectroscopy. 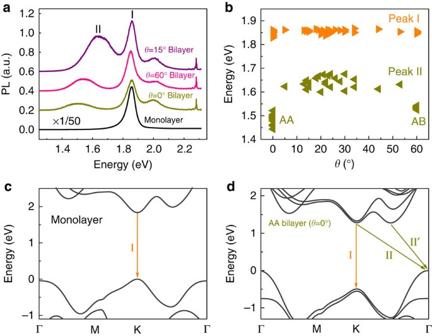Figure 2: Probing interlayer electronic coupling in twisted MoS2bilayers. (a) Photoluminescence (PL) spectra of MoS2monolayer and bilayers with twist angles ofθ=0°, 15° and 60°. (b) Dependence of PL peak energies on the twist angle for 44 MoS2bilayers. The peak I energy is almost identical for all bilayers. The peak II energy is lowest for AA- and AB-stacked bilayers, and is higher but at a nearly constant value for other twist angles. (c,d) Calculated local density approximation (LDA) Kohn–Sham band structure of a MoS2monolayer (c) and of the most energetically favourable AA-stacked bilayer (d). Transition I is associated with the K-valley direct bandgap (peak I in PL spectra). The indirect bandgap transitions II and II′ have nearly degenerate energy and either may be associated with the peak II in the PL spectra. Figure 2a shows the typical PL spectra of a MoS 2 monolayer and bilayers with twist angles of θ =0°, 15° and 60°. The monolayer PL spectrum features a prominent peak of ~1.85 eV (peak I) that corresponds to the exciton transition at the K-valley of the Brillouin zone ( Fig. 2c ). For all bilayers, the direct exciton transition at the K-valley of the original monolayer Brillouin zone (peak I) remains, but its PL intensity decreases significantly (to ~1/50 of the monolayer PL). In addition, a new peak at lower energy (peak II) appears. The emergence of this new peak II corresponds to an indirect bandgap resulting from the interlayer electronic coupling, in which the doubly degenerate valence band splits into two branches near the Γ point and the upper branch rises to an energy higher than the valence band at the K point in the monolayer Brillouin zone ( Fig. 2d ). Therefore, the indirect bandgap (peak II) energy reflects directly the interlayer electronic coupling strength: the lower the indirect bandgap, the stronger the coupling strength. To investigate the evolution of electronic coupling in twisted bilayers in more detail, we systematically studied 44 MoS 2 bilayers with various twist angles. Figure 2b displays the transition energies of peaks I and II in all measured bilayers that exhibit interesting dependence on the twist angle. In contrast to a virtually unchanged peak I energy (direct exciton transition), the peak II energy (indirect transition) is lowest for perfect registered (that is, AA- and AB-stacked) bilayers, and has a higher but nearly constant value for all other twist angles. This means that the interlayer electronic coupling is significant for all twist angles, but is the strongest in AA- or AB-stacked MoS 2 bilayers. Figure 2: Probing interlayer electronic coupling in twisted MoS 2 bilayers. ( a ) Photoluminescence (PL) spectra of MoS 2 monolayer and bilayers with twist angles of θ =0°, 15° and 60°. ( b ) Dependence of PL peak energies on the twist angle for 44 MoS 2 bilayers. The peak I energy is almost identical for all bilayers. The peak II energy is lowest for AA- and AB-stacked bilayers, and is higher but at a nearly constant value for other twist angles. ( c , d ) Calculated local density approximation (LDA) Kohn–Sham band structure of a MoS 2 monolayer ( c ) and of the most energetically favourable AA-stacked bilayer ( d ). Transition I is associated with the K-valley direct bandgap (peak I in PL spectra). The indirect bandgap transitions II and II′ have nearly degenerate energy and either may be associated with the peak II in the PL spectra. Full size image Interlayer mechanical couplings evolution in MoS 2 bilayers In addition to the electronic bandgaps, we investigated the evolution of phonon vibrations in twisted MoS 2 bilayers using Raman scattering spectroscopy. 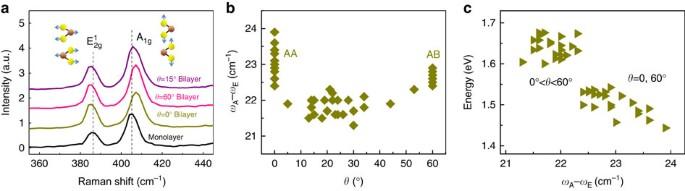Figure 3: Probing interlayer mechanical coupling in twisted MoS2bilayer. (a) Raman spectra of a MoS2monolayer and bilayers with twist angles ofθ=0°, 15° and 60°. (b) Raman peak separation between the A1gand E2g1(ωA−ωE) in MoS2bilayers of different twist angles, which is the largest for AA or AB stacking and nearly a constant for other twist angles. (c) The relation between peak II inFig. 2band Raman peak separation. The data collapse onto a linear line, indicating an intrinsic correlation between electronic and mechanical coupling. Figure 3a shows the typical Raman spectra of a MoS 2 monolayer and bilayers with twist angles of θ =0°, 15° and 60°. Two prominent peaks are observed in the range of 360–440 cm −1 and are assigned to the in-plane E 2g 1 and out-of-plane A 1g phonon modes ( Fig. 3a , inset), respectively. Previous Raman studies suggest that interlayer coupling softens the E 2g 1 mode through an enhanced dielectric screening dependent on the layer number, whereas it stiffens the A 1g mode [32] , [33] . Indeed, for bilayers, the E 2g 1 peak shows a constant redshift, whereas the A 1g peak exhibits a twist angle-dependent blueshift. Therefore, the separation between these two peaks ( ω A − ω E ) characterizes the effective interlayer mechanical coupling strength: the further the separation, the stronger the coupling strength. Figure 3b shows the Raman peak separation in 44 MoS 2 bilayers with respect to the twist angle. Interestingly, the mechanical coupling shows a pattern very similar to that of the electronic coupling as in Fig. 2b : AA or AB stacking has the strongest coupling and the other twist angles have weaker but constant coupling. Figure 3: Probing interlayer mechanical coupling in twisted MoS 2 bilayer. ( a ) Raman spectra of a MoS 2 monolayer and bilayers with twist angles of θ =0°, 15° and 60°. ( b ) Raman peak separation between the A 1g and E 2g 1 ( ω A − ω E ) in MoS 2 bilayers of different twist angles, which is the largest for AA or AB stacking and nearly a constant for other twist angles. ( c ) The relation between peak II in Fig. 2b and Raman peak separation. The data collapse onto a linear line, indicating an intrinsic correlation between electronic and mechanical coupling. Full size image Theory for electronic bandgap evolution in MoS 2 bilayers In order to understand the unusual evolution of interlayer coupling in twisted MoS 2 bilayers, we perform ab initio calculations on the structural energy and band structures of MoS 2 bilayers from density functional theory within the local density approximation (LDA). A supercell approach is used to describe the twisted bilayers, with the crystalline alignment of the top layer oriented at a commensurate angle with respect to the bottom layer. θ =0°, 60° and four intermediate commensurate angles ( θ ~13°, 22°, 38° and 47°) are studied in our calculations ( Fig. 4a ). When θ =0° (AA) or 60° (AB), there are three high-symmetry stacking configurations: the S atoms in the top layer are placed above (1) the Mo atoms (AA 1 and AB 1 ), (2) the hexagonal centres (AA 2 and AB 2 ),or (3) the S atoms in the bottom layer (AA 3 and AB 3 ). As the AA 1 and the AA 2 configurations are related by spatial inversion, we use AA 1 to denote these two equivalent structures. Among these high-symmetry configurations, AA 1 and AB 1 have the lowest energy and are presumably the most stable ( Supplementary Fig. 1 ). For the four twisted configurations, there are no high-symmetry configurations, and the atoms in the two layers have nearly random relative distributions. Our calculated Kohn–Sham K-valley direct bandgaps (that is, bandgaps responsible for the direct optical transition originating from the K-valley of the first Brillouin zone of a monolayer MoS 2 unit cell) and the indirect bandgaps (that is, the smallest bandgap between the valence band top and the conduction band minimum) for AA 1 , AB 1 and the four twisted configurations are shown in Fig. 4b . We find that the trend in bandgap variation with the twist angle matches well with the experimental observation in Fig. 2b : The K-valley direct bandgap remains largely unchanged, but the indirect bandgap is much smaller in AA- and AB-stacked bilayers compared with all other twist angles. We note that the Kohn–Sham bandgaps should not be directly compared with the measured optical bandgaps because of the neglect of the quasiparticle self-energy and electron-hole interaction effect [17] ; however, these effects tend to cancel each other in the transition energies. The trends in the twist angle dependence should be correct. 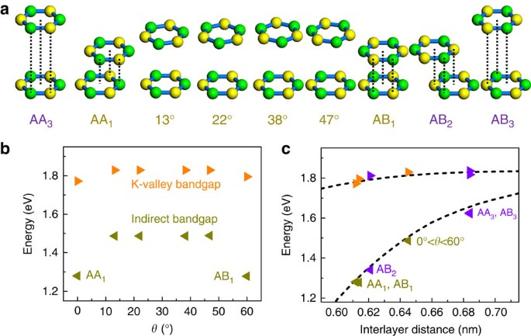Figure 4: Structural and bandgap calculations of MoS2bilayers. (a) Schematics of MoS2bilayers with AA, AB and different twisted configurations. Mo atoms are shown as green spheres; two S atoms of the same horizontal position are presented by one yellow sphere. Interlayer distance variations are exaggerated for illustration. The interlayer separation is ~0.61 nm for AA1and AB1stacking, ~0.62 nm for AB2stacking, ~0.68 nm for AA3and AB3stacking and~0.65 nm for the four twisted bilayers. (b) Calculated values for the Kohn–Sham K-valley direct bandgap (orange) and indirect bandgap (dark yellow) for the energetically favourable structures at each twist angle. (c) The calculated Kohn–Sham bandgap as a function of the interlayer distance for different stacking configurations (symbols). The dashed curve shows the bandgap values for AA1stacking with artificially varied interlayer separation. Their comparison indicates that the electronic coupling in MoS2bilayer is largely determined by the interlayer separation and does not depend explicitly on the horizontal registration of the two layers. Figure 4: Structural and bandgap calculations of MoS 2 bilayers. ( a ) Schematics of MoS 2 bilayers with AA, AB and different twisted configurations. Mo atoms are shown as green spheres; two S atoms of the same horizontal position are presented by one yellow sphere. Interlayer distance variations are exaggerated for illustration. The interlayer separation is ~0.61 nm for AA 1 and AB 1 stacking, ~0.62 nm for AB 2 stacking, ~0.68 nm for AA 3 and AB 3 stacking and~0.65 nm for the four twisted bilayers. ( b ) Calculated values for the Kohn–Sham K-valley direct bandgap (orange) and indirect bandgap (dark yellow) for the energetically favourable structures at each twist angle. ( c ) The calculated Kohn–Sham bandgap as a function of the interlayer distance for different stacking configurations (symbols). The dashed curve shows the bandgap values for AA 1 stacking with artificially varied interlayer separation. Their comparison indicates that the electronic coupling in MoS 2 bilayer is largely determined by the interlayer separation and does not depend explicitly on the horizontal registration of the two layers. Full size image Theory for interlayer distance evolution in MoS 2 bilayers We further examine the evolution of the calculated interlayer distance (defined by the averaged Mo–Mo interlayer separation). A strong variation of the interlayer distance on the stacking configuration is found, as illustrated in an exaggerated fashion in Fig. 4a (see detailed value in Table 1 ). The higher energy AA 3 and AB 3 configurations have the largest interlayer distance of ~0.68 nm; the two energetically favourable AA 1 , and AB 1 configurations are found to have the smallest interlayer distance of ~0.61 nm, and all the twisted configurations have almost identical interlayer distances at~0.65 nm. If we only focus on the lower energy configurations (AA 1 , AB 1 and the four twisted configurations), this trend in interlayer distance evolution with twist angle is similar to the evolution of the indirect bandgap ( Fig. 4b ). Table 1 Calculated interlayer distance of MoS 2 bilayers in different configurations. Full size table The configuration-dependent interlayer distance in bilayer MoS 2 can be understood physically by steric effects that arise from the fact that each atom occupies a certain amount of space that strongly repulse other atoms owing to a significant energy cost from overlapping electron clouds. Between two vertically stacked MoS 2 layers, the only interlayer adjacent atoms are S atoms. In the energetically unfavourable AA 3 or AB 3 stacking configurations, the S atoms of the top layer sit directly on the S atoms of the bottom layer in an eclipsed fashion, leading to a strong repulsion and the largest interlayer distance. In the energetically favourable AA 1 or AB 1 stacking configurations, on the other hand, the S atoms of the top layer sit on the trigonal vacancies of the S atoms of the bottom layer in a staggered fashion, resulting in reduced repulsion and the smallest interlayer distance. For other twist angles, the S atoms of the top layer sit nearly randomly relative to the S atoms of the bottom layer, and therefore, the interlayer distance is constant and roughly at the average of that of the most stable AA 1 (AB 1 ) and unstable AA 3 (AB 3 ) stacking configurations. Consequently, the variation in interlayer distance has a simple geometric origin, which is determined by the lateral registration of adjacent S layers. Such steric effects determine the interlayer distance that in turn modifies both the interlayer electronic and mechanical coupling strengths. This explains why these two types of coupling share similar evolutionary trends with twist angle and why they are almost linearly related ( Fig. 3c ). Interestingly, if we examine separately the explicit dependence of the electronic coupling (and the corresponding indirect bandgap energy) on the interlayer vertical separation and horizontal registration, only the former has a significant effect. For example, we can artificially vary the interlayer distance of the AA 1 -stacked bilayer in our ab initio calculation and calculate the resulting changes in the direct and indirect Kohn–Sham bandgaps (dashed curves in Fig. 4c ). Surprisingly, the bandgap versus interlayer distance relation for different stacking configurations (symbols in Fig. 4c ) all lie on the dashed curves, which are from the AA 1 configuration at different separation. It shows that in MoS 2 bilayers, the interlayer coupling strength of the electronic states near the band edges depends only explicitly on the interlayer distance, but not on the relative horizontal lattice alignment. (We note that there is an implicit dependence because the interlayer separation varies with the horizontal lattice registration). We notice that the PL peak II can vary significantly for AA- and AB-stacked bilayers. Presumably, it arises from uncontrollable interlayer distance variation in the CVD-grown bilayers. For example, the thermal expansion coefficient of MoS 2 is one order of magnitude larger than the fused silica substrate that can induce a mechanical strain in the bilayer and lead to relative slipping between the two layers. This will result in a change in average distance for AA- and AB-stacked bilayers and variations of the indirect bandgap, but has little effect on bilayers with twisting angle between 0 and 60°. Our discovery indicates that the steric repulsion effects, which have been extensively studied in surface reactions and nano-bio interfaces, also have an important role in understanding the electronic and vibrational properties of vdW-coupled 2D atomic layers. Such steric effects have been largely overlooked in previous studies of graphene systems [1] , [2] , [3] , [4] , [5] , [6] . Our calculations show that the steric effects in 2D atomic layers strongly depend on the atomic size and the in-plane atom–atom distance. Comparing MoS 2 with graphene, it was found that not only is the size of S atoms bigger than the size of C atoms but also the in-plane S–S distance (0.32 nm) much larger than the in-plane C–C distance (0.14 nm). As a result, the steric effect is ~3 times stronger in MoS 2 bilayers than graphene bilayers. Still, steric effects are present in graphene bilayers in which the interlayer distance of Bernal-stacked graphene bilayers is 0.01 nm smaller than that of other twisted bilayers ( Supplementary Table 1 ). In conclusion, we investigate the interlayer coupling evolution in twisted MoS 2 bilayers and find that the change in both electronic and mechanical interlayer coupling is relatively constant at twist angles between 0 and 60°, and becomes strongest for twist angle at 0°(AA stacking) and at 60°(AB stacking). In particular, we identify the importance of the varying interlayer distance in vdW-coupled 2D atomic-layered materials. The interlayer distance can potentially be tuned through material design or external pressure. This tunability may expand the range of optical, mechanical and electrical properties of these 2D materials for device applications. Growth of twisted MoS 2 bilayers We grew MoS 2 bilayers by CVD method on mica, fused silica or SiO 2 /Si substrate using MoO 3 and S powder as precursors. The substrate was loaded into a 1-inch CVD furnace and placed above a crucible containing 20 mg of MoO 3 (≥99.5%, Sigma-Aldrich). Another crucible containing 7 mg of S (≥99.5%, Sigma-Aldrich) was placed 12 cm upstream from the sample. The CVD process was performed under ambient pressure while flowing ultrahigh-purity nitrogen. The recipe is as follows: sit at 105 °C with 500 sccm for 1 h, ramp to 700 °C at 15 °C min −1 with 10–15 sccm N 2 , sit at 700 °C for 5–10 min and then cool down naturally with 500 sccm gas flow. The ratio of MoS 2 bilayer to monolayer increases with the growth time. Bilayers with yield as high as 30% can be achieved when performing 10 min growth under 700 °C. In general, the yield of AA-stacked bilayer of θ =0° is the highest (~85%), followed by AB-stacked bilayer of θ =60° (~10%). Difference reflection spectra measurements A supercontinuum laser (470–1,800 nm) was used as the light source. We focused the supercontinuum to a diameter of ~2 μm on the sample and analysed the reflected light with a spectrograph equipped with an array charge-coupled device detector. Two sets of reflection spectra with the MoS 2 monolayers or bilayers inside the laser beam ( I inside ) and outside the beam ( I outside ) were taken, and the final difference spectrum was obtained as Δ R / R =( I inside − I outside )/ I outside . SHG measurements A femtosecond laser (ATSEVA TiF-100F laser, 80 MHz repetition rate, wavelength at 800 nm and pulse duration of 100 fs) was used as the light source. We used 20 mW linearly polarized light focused to a diameter of ~5 μm for excitation, and collected the SHG signal using a spectrometer coupled with a charge-coupled device. PL and Raman spectra measurements They were taken by a Horiba HR800 system with laser excitation wavelength of 532 nm. The laser is focused to a diameter of ~1 μm and has a power of ~1 mW. Ab initio calculations Ab initio calculations of twisted MoS 2 bilayers were performed using density functional theory in the LDA implemented in the Quantum Espresso package [34] . A supercell arrangement was used with the cell dimension in the out-of-plane direction set at 20 Å to avoid interactions between the MoS 2 bilayer and its periodic images. We use norm-conserving pseudopotentials with a plane-wave energy cutoff of 140 Ry. The structures were fully relaxed until the force on each atom is <0.01 eV/Å. Spin-orbit coupling was not included in our calculations. We also carried out the theoretical calculations for different bilayer configurations using the Perdew–Burke–Ernzerhof exchange-correlation functional with dispersion correction (PBE-D). The interlayer distances obtained with the method are almost identical to that from LDA calculations ( Table 1 ). Consequently, the evolution of bandgaps calculated using the PBE-D method shows a similar trend as that obtained from LDA calculations ( Supplementary Fig. 2 ). How to cite this article : Liu, K. et al . Evolution of interlayer coupling in twisted molybdenum disulfide bilayers. Nat. Commun. 5:4966 doi: 10.1038/ncomms5966 (2014).